Automated home-cage behavioural phenotyping of mice Neurobehavioural analysis of mouse phenotypes requires the monitoring of mouse behaviour over long periods of time. In this study, we describe a trainable computer vision system enabling the automated analysis of complex mouse behaviours. We provide software and an extensive manually annotated video database used for training and testing the system. Our system performs on par with human scoring, as measured from ground-truth manual annotations of thousands of clips of freely behaving mice. As a validation of the system, we characterized the home-cage behaviours of two standard inbred and two non-standard mouse strains. From these data, we were able to predict in a blind test the strain identity of individual animals with high accuracy. Our video-based software will complement existing sensor-based automated approaches and enable an adaptable, comprehensive, high-throughput, fine-grained, automated analysis of mouse behaviour. Automated quantitative analysis of mouse behaviour will have a significant role in comprehensive phenotypic analyses—both on the small scale of detailed characterization of individual gene mutants and on the large scale of assigning gene function across the entire mouse genome [1] . One key benefit of automating behavioural analysis arises from inherent limitations of human assessment, namely, cost, time and reproducibility. Although automation in and of itself is not a panacea for neurobehavioural experiments [2] , it allows for addressing an entirely new set of questions about mouse behaviour and to conduct experiments on time scales that are orders of magnitude larger than those traditionally assayed. For example, reported tests of grooming behaviour span time scales of minutes [3] , [4] , whereas an automated analysis will allow for analysis of this behaviour over hours or even days and weeks. Indeed, the significance of alterations in home-cage behaviour has recently gained attention as an effective means of detecting perturbations in neural circuit function—both in the context of disease detection and more generally to measure food consumption and activity parameters [5] , [6] , [7] , [8] , [9] , [10] . Previous automated systems (see refs 8 , 9 , 11 , 12 and Supplementary Note ) rely mostly on the use of simple detectors such as infrared beams to monitor behaviour. These sensor-based approaches tend to be limited in the complexity of the behaviour that they can measure, even in the case of costly commercial systems using transponder technologies [13] . Although such systems can be used effectively to monitor locomotor activity and perform operant conditioning, they cannot be used to study home-cage behaviours such as grooming, hanging, jumping and smaller movements (termed 'micromovements' below). Visual analysis is a potentially powerful complement to these sensor-based approaches for the recognition of such fine animal behaviours. Advances in computer vision and machine learning over the last decade have yielded robust computer vision systems for the recognition of objects [14] , [15] and human actions (see Moeslund et al . [16] for review). In fact, the use of vision-based approaches is already bearing fruit for the automated tracking [17] , [18] , [19] and recognition of behaviours in insects [20] , [21] . Several open-source and commercial computer vision systems for the recognition of mouse behaviour have also been developed (see study by Xue and Henderson [22] , and Dollar et al . [23] and Supplementary Note ). However, these systems are not widely used, exhibit similar limitations to sensor-based approaches and/or are cost prohibitive. In this paper, we describe a trainable, general-purpose, automated and potentially high-throughput system for the behavioural analysis of mice in their home cage. Developed from a computational model of motion processing in the primate visual cortex [24] , [25] , the computer system is trained with labelled examples with manually annotated behaviours of interest and used to automatically analyse new recordings containing hours of freely behaving animals. As a proof of concept, we trained the system on common mouse behaviours and demonstrated that the resulting system performs on par with humans for the scoring of these behaviours. Using the resulting system, we analysed the home-cage behaviour of several mouse strains, including the commonly used strains C57BL/6J, DBA/2J, the BTBR strain that displays autistic-like behaviours, as well as a wild-derived strain CAST/EiJ. We characterize differences in the behaviours of these strains and use these profiles to predict the strain type of an animal. Our system (available as Supplementary Software ) consists of three separate modules: (I) a video database, (II) a feature computation module and (III) a classification module. The latest software can be found at http://cbcl.mit.edu/software-datasets/hueihan/index.html . Video database We video recorded a large database of video sequences of singly housed mice in their home cages from an angle perpendicular to the side of the cage (see Fig. 1 for examples of video frames) using a consumer grade camcorder. To create a robust recognition system, we varied the lighting conditions by placing the cage in different positions with respect to the overhead lighting. In addition, we used many mice of different size, gender and coat colour. We considered eight behaviours of interest, which included drinking, eating, grooming, hanging, rearing, walking, resting and micromovements of the head. Several investigators were trained to score mouse behaviour using two different scoring techniques. 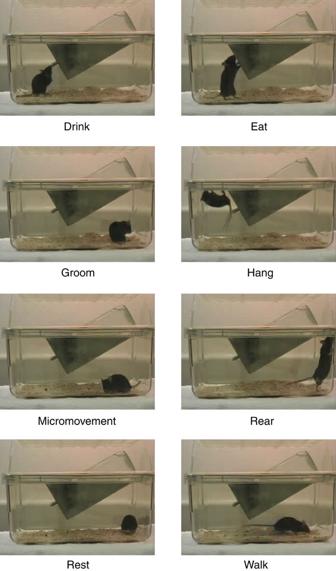Figure 1: Home-cage behaviours for training the system. Snapshots taken from representative videos for the eight home-cage behaviours of interest. Figure 1: Home-cage behaviours for training the system. Snapshots taken from representative videos for the eight home-cage behaviours of interest. Full size image The first set of annotations, denoted the 'clipped database' ( http://serre-lab.clps.brown.edu/projects/mouse_behavior/ ), included only clips scored with very high stringency, seeking to annotate only the best and most exemplary instances of particular behaviours. A pool of eight annotators ('Annotator group 1') manually hand-scored more than 9,000 short clips, each containing a unique annotation. To avoid errors, this database was then curated by one of the annotators who watched all 9,000 clips again, retaining only the most unambiguous assessments, leaving 4,200 clips (262,360 frames corresponding to about 2.5 h) from 12 distinct videos (recorded at 12 separate sessions) to train and tune the feature computation module of the proposed system, as described below. The second set of annotations, called the 'full database', involved labelling every frame (with less stringency than in the 'clipped database') for 12 unique videos (different from the 12 videos used in the 'clipped database') corresponding to over 10 h of continuously annotated video ( http://serre-lab.clps.brown.edu/projects/mouse_behavior/ ). Again, two sets of annotators were used to correct mistakes and ensure that the annotation style was consistent throughout the whole database. This database was used to train and test the classification module of the computer system. The distribution of behaviour labels for the 'clipped database' and the 'full database' is shown in Supplementary Figures S1a–b and Supplementary Figures S1c–d, respectively. Computation and evaluation of motion and position features The architecture used here to preprocess raw video sequences ( Fig. 2a,b ) and extract motion features ( Fig. 2c ) is adapted from previous work for the recognition of human actions and biological motion [25] . To speed up the system, the computation of the motion features was limited to a subwindow centred on the animal ( Fig. 2b ), the location of which can be computed from the foreground pixels obtained by subtracting off the video background ( Fig. 2a ). For a static camera as used here, the video background can be well approximated by a median frame in which each pixel value corresponds to the median grey value computed over all frames for that pixel location (day and night frames under red lights were processed in separate videos). 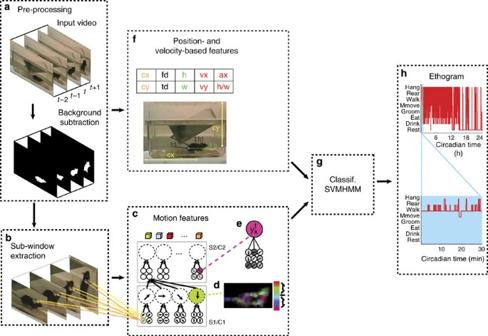Figure 2: Overview of the proposed system for monitoring the home-cage behaviour of mice. The computer vision system consists of a feature computation module (a–f) and a classification module (g). (a) A background subtraction procedure is first applied to an input video to compute a foreground mask for pixels belonging to the animal versus the cage. (b) A subwindow centred on the animal is cropped from each video frame based on the location of the mouse (seeSupplementary Method). Two types of features are then computed: (c) space-time motion features and (f) position- and velocity-based features. To speed up the computation, motion features are extracted from the subwindow (b) only. These motion features are derived from combinations of the response of afferent units that are tuned to different directions of motion as found in the mammalian primary visual cortex (d,e). (f) Position- and velocity-based features are derived from the instantaneous location of the animal in a cage. These features are computed from a bounding box tightly surrounding the animal in the foreground mask. (g) The output of this feature computation module consists of 310 features per frame that are then passed to a statistical classifier, SVMHMM (Hidden Markov Model Support Vector Machine), to reliably classify every frame of a video sequence into a behaviour of interest. (h) An ethogram of the sequence of labels predicted by the system from a 24-h continuous recording session for one of the CAST/EiJ mice. The red panel shows the ethogram for 24 h, and the light blue panel provides a zoomed version corresponding to the first 30 min of recording. The animal is highly active, as it was just placed in a new cage before starting the video recording. The animal's behaviour alternates between 'walking', 'rearing' and 'hanging' as it explores the new cage. Figure 2: Overview of the proposed system for monitoring the home-cage behaviour of mice. The computer vision system consists of a feature computation module ( a – f ) and a classification module ( g ). ( a ) A background subtraction procedure is first applied to an input video to compute a foreground mask for pixels belonging to the animal versus the cage. ( b ) A subwindow centred on the animal is cropped from each video frame based on the location of the mouse (see Supplementary Method ). Two types of features are then computed: ( c ) space-time motion features and ( f ) position- and velocity-based features. To speed up the computation, motion features are extracted from the subwindow ( b ) only. These motion features are derived from combinations of the response of afferent units that are tuned to different directions of motion as found in the mammalian primary visual cortex ( d , e ). ( f ) Position- and velocity-based features are derived from the instantaneous location of the animal in a cage. These features are computed from a bounding box tightly surrounding the animal in the foreground mask. ( g ) The output of this feature computation module consists of 310 features per frame that are then passed to a statistical classifier, SVMHMM (Hidden Markov Model Support Vector Machine), to reliably classify every frame of a video sequence into a behaviour of interest. ( h ) An ethogram of the sequence of labels predicted by the system from a 24-h continuous recording session for one of the CAST/EiJ mice. The red panel shows the ethogram for 24 h, and the light blue panel provides a zoomed version corresponding to the first 30 min of recording. The animal is highly active, as it was just placed in a new cage before starting the video recording. The animal's behaviour alternates between 'walking', 'rearing' and 'hanging' as it explores the new cage. Full size image The computation of motion features is based on the organization of the dorsal stream of the visual cortex, which has been linked to the processing of motion information (see study by Born and Bradley [26] for a recent review). Details about the implementation are provided in the Supplementary Methods . A hallmark of the system is its hierarchical architecture: The first processing stage corresponds to an array of spatio-temporal filters tuned to four different directions of motion and modelled after motion-sensitive (simple) cells in the primary visual cortex (V1) [27] (S1/C1 layers, Fig. 2d ). The architecture then extracts space-time motion features centred at every frame of an input video sequence via multiple processing stages, whereby features become increasingly complex and invariant with respect to two-dimensional transformations as one moves up the hierarchy. These motion features are obtained by combining the response of V1-like afferent motion units that are tuned to different directions of motion ( Fig. 2e ). The output of this hierarchical preprocessing module consists of a dictionary of about 300 space-time motion features (S2/C2 layers, Fig. 2e ) that are obtained by matching the output of the S1/C1 layers with a dictionary of motion-feature templates. This basic dictionary of motion-feature templates corresponds to discriminative motion features that are learnt from a training set of videos containing labelled behaviours of interest (the 'clipped database'), through a feature selection technique. To optimize the performance of the system for the recognition of mouse behaviours, several key parameters of the model were adjusted. The parameters of the spatio-temporal filters in the first stage (e.g., their preferred speed tuning and direction of motion, the nature of the nonlinear transfer function used, the video resolution and so on) were adjusted so as to maximize performance on the 'clipped database'. To evaluate the quality of these motion features for the recognition of high-quality unambiguous behaviours, we trained and tested a multiclass Support Vector Machine (SVM) on single isolated frames from the 'clipped database' using the all-pair multiclass classification strategy. This approach does not rely on the temporal context of measured behaviours beyond the computation of low-level motion signals and classifies each frame independently. On the 'clipped database', we find that such a system leads to 93% accuracy (as the percentage of correctly predicted clips, chance level is 12.5% for an eight-class classification), which is significantly higher than the performance of a representative computer vision system [23] (81%) trained and tested under the same conditions (see Supplementary Methods ). Performance was estimated on the basis of a leave-one-video-out procedure, whereby clips from all except one video are used to train the system, whereas performance is evaluated on the clips from the remaining video. The procedure was repeated for all videos; we report the overall accuracy. This suggests that the representation provided by the dictionary of motion-feature templates is suitable for the recognition of the behaviours of interest even under conditions in which the global temporal structure (i.e., the temporal structure beyond the computation of low-level motion signals) of the underlying temporal sequence is discarded. In addition to the motion features described above, we computed an additional set of features derived from the instantaneous location of the animal in the cage ( Fig. 2f ). Position- and velocity-based measurements were estimated on the basis of the two-dimensional coordinates ( x , y ) of the foreground pixels ( Fig. 2a ) for every frame. These included the position and aspect ratio of the bounding box around the animal (indicating whether the animal is in a horizontal or vertical posture), the distance of the animal to the feeder, as well as its instantaneous velocity and acceleration. Figure 2f illustrates some of the key features used (see Supplementary Table S1 for a complete list). Classification module The reliable phenotyping of an animal requires more than the mere detection of stereotypical non-ambiguous behaviours. In particular, the present system aims at classifying every frame of a video sequence, even for those frames that are ambiguous and difficult to categorize. For this challenging task, the temporal context of a specific behaviour becomes an essential source of information; thus, learning an accurate temporal model for the recognition of actions becomes critical (see Supplementary Fig. S2 for an illustration). In this study we used a Hidden Markov Model Support Vector Machine (SVMHMM, Fig. 2g ) [28] , [29] , which is an extension of the SVM classifier for sequence tagging. This temporal model was trained on the 'full database' as described above, which contains manually labelled examples of about 10 h of continuously scored video sequences from 12 distinct videos. Assessing the accuracy of the system is a critical task. Therefore, we made two comparisons: (I) between the resulting system and commercial software (HomeCageScan 2.0, CleverSys Inc.) for mouse home-cage behaviour classification and (II) between the system and human annotators. The level of agreement between human annotators sets a benchmark for the system performance, as the system relies entirely on human annotations to learn to recognize behaviours. To evaluate the agreement between two sets of labellers, we asked a set of four human annotators ('Annotator group 2') independent from 'Annotator group 1' to annotate a subset of the 'full database'. This subset (denoted 'set B') corresponds to many short random segments from the 'full database'; each segment is about 5–10 min in length and they add up to a total of 1.6 h of annotated video. Supplementary Figure S1d shows the corresponding distribution of labels for 'set B' and confirms that 'set B' is representative of the 'full database' ( Supplementary Fig. S1c ). Performance was estimated using a leave-one-video-out procedure, whereby all but one of the videos was used to train the system, and performance was evaluated on the remaining video. The procedure was repeated n =12 times for all videos and the performance averaged. We found that our system achieves 77.3% agreement with human labellers on 'set B' (averaged across frames), a result substantially higher than the HomeCageScan 2.0 (60.9%) system and on par with humans (71.6%), as shown in Table 1 . For all the comparisons above, the annotations made by the 'Annotator group 1' were used as ground truth to train and test the system because these annotations underwent a second screening and were therefore more accurate than the annotations made by the 'Annotator group 2'. The second set of annotations made by the 'Annotator group 2' on 'set B' was only used for measuring the agreement between independent human annotators. It is therefore possible for a computer system to appear more 'accurate' than the second group of annotators, which is in fact what we observed for our system. Table 1 also shows the comparison between the system and commercial software on the 'full database'. Table 1 Accuracy of the system. 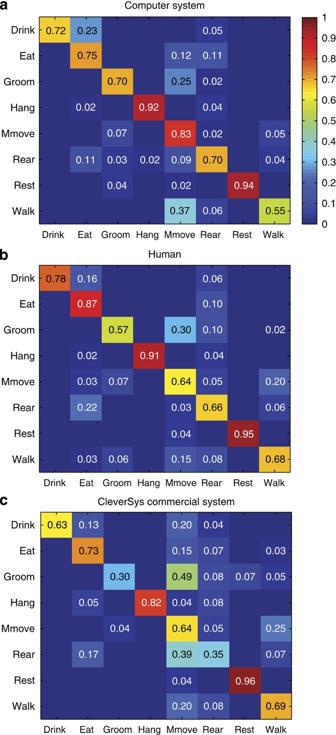Figure 3: Confusion matrix of the system. Confusion matrices evaluated on the doubly annotated 'set B' to compare the agreement between (a) the system and human scoring, (b) human to human scoring and (c) the CleverSys system to human scoring. Each entry (x,y) in the confusion matrix is the probability with which an instance of a behaviourx(along rows) is classified as typey(along column), and which is computed as (number of frames annotated as typexand classified as typey)/(number of frames annotated as typex). As a result, values sum to a value of 1 in each row. The higher probabilities along the diagonal and the lower off-diagonal values indicate successful classification for all categories. Using the annotations made by the 'Annotator group 1' as ground truth, the confusion matrix was obtained for measuring agreement between ground truth (row) with system (computer system), with the 'Annotator group 2' (human) and with baseline software (CleverSys commercial system). For a less cluttered visualization, entries with values less than 0.01 are not shown. The colour bar indicates the percentage agreement, with more intense shades of red indicating agreements close to 100% and lighter shades of blue indicating small percentages of agreement. Full size table Figure 3 shows the confusion matrices between the computer system and 'Annotator group 1' ( Fig. 3a ), between 'Annotator group 1' and 'Annotator group 2' ( Fig. 3b ), as well as between the HomeCageScan system and 'Annotator group 1' ( Fig. 3c ). A confusion matrix is one way to visualize the agreement between two entities, wherein each entry ( x , y ) of the matrix represents the probability that the first entity (say 'Annotator group 1') will label a specific behaviour as x and the second entity (say the computer system ) as y . For instance, two entities with perfect agreement would exhibit a 1 value along every entry along the diagonal and 0 everywhere else. In Figure 3a for example, the matrix value along the fourth row and fourth column indicates that the computer system correctly classifies 92% of the 'hanging' behaviours as labelled by a human observer, whereas 8% of the behaviours are incorrectly classified as 'eating' (2%), rearing (5%) or others (less than 1%). These numbers are also reflected in the colour codes used, with red/blue corresponding to better/worse levels of agreement. We also observed that adding the position- and velocity-based features led to an improvement in the system's ability to discriminate between visually similar behaviours and for which the location of the animal in the cage provides critical information (see Supplementary Methods and Supplementary Fig. S3 ). For example, drinking (versus eating) occurs at the water bottle spout, whereas hanging (versus rearing) mice have at least two limbs off the ground. Examples of automated scoring of videos by the system are available as Supplementary Movies 1 and 2 . Figure 3: Confusion matrix of the system. Confusion matrices evaluated on the doubly annotated 'set B' to compare the agreement between ( a ) the system and human scoring, ( b ) human to human scoring and ( c ) the CleverSys system to human scoring. Each entry ( x , y ) in the confusion matrix is the probability with which an instance of a behaviour x (along rows) is classified as type y (along column), and which is computed as (number of frames annotated as type x and classified as type y )/(number of frames annotated as type x ). As a result, values sum to a value of 1 in each row. The higher probabilities along the diagonal and the lower off-diagonal values indicate successful classification for all categories. Using the annotations made by the 'Annotator group 1' as ground truth, the confusion matrix was obtained for measuring agreement between ground truth (row) with system (computer system), with the 'Annotator group 2' (human) and with baseline software (CleverSys commercial system). For a less cluttered visualization, entries with values less than 0.01 are not shown. The colour bar indicates the percentage agreement, with more intense shades of red indicating agreements close to 100% and lighter shades of blue indicating small percentages of agreement. Full size image How scalable is the proposed approach to new behaviours? How difficult would it be to train the proposed system for the recognition of new behaviours or environments (e.g., outside the home cage and/or using a camera from a different viewpoint?). The main aim of this study was to build a system that generalizes well with many different laboratory settings. For this reason, we collected and annotated a large data set of videos. Sometimes, however, it might be advantageous to train a more 'specialized' system very quickly from very few training examples. To investigate this issue, we systematically evaluated the performance of the system as a function of the amount of training videos available for training. 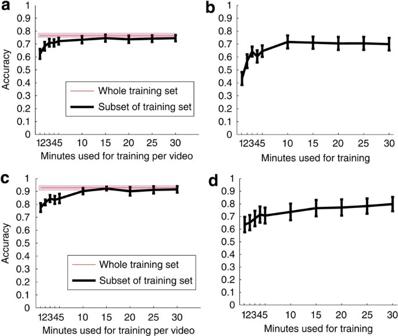Figure 4: Training the system with varying numbers of examples. For this leave-one-video-out experiment, the system accuracy is computed as a function of the amount of video data (in minutes/video) used for training the system. For each leave-one-out trial, the system is trained on a representative set of videos and tested on the full length of the video left out. A representative set consisting ofx1-min segments is manually selected such that the total time of each of the eight behaviours is roughly the same. (a) Average accuracy and standard error across the 12 leave-one-out runs on the 'full database'. (b) Average accuracy and standard error across the 12 runs on the 'full database'. (c) Average accuracy and standard error across the 13 leave-one-out runs on the 'wheel-interaction database'. We also perform the training/testing on the same video: a representative set of video segments is selected from the first 30 min of each video for training; testing is carried out on the remaining of the video from the 30th minute to the end of the same video. System accuracy is computed as a function of the amount of video data (in minute) used for training. (d) Average accuracy and standard error across the 13 runs on the 'wheel-interaction database'. Figure 4a shows that a relatively modest amount of training data (that is, as little as 2 min of labelled video for each of the 11 training videos) is indeed sufficient for robust performance (correspond to 90% of the performance obtained using 30min of annotations for each video). In addition, in such cases in which generalization is not required, an efficient approach would be to train the system on the first few minutes of a video and then let the system complete the annotation on the rest of the video. Figure 4b shows that by using a representative set of only 3 min of video data, the system is already able to achieve 90% of its peak level. Near peak performance can be achieved using 10 min of a single video for training. Figure 4: Training the system with varying numbers of examples. For this leave-one-video-out experiment, the system accuracy is computed as a function of the amount of video data (in minutes/video) used for training the system. For each leave-one-out trial, the system is trained on a representative set of videos and tested on the full length of the video left out. A representative set consisting of x 1-min segments is manually selected such that the total time of each of the eight behaviours is roughly the same. ( a ) Average accuracy and standard error across the 12 leave-one-out runs on the 'full database'. ( b ) Average accuracy and standard error across the 12 runs on the 'full database'. ( c ) Average accuracy and standard error across the 13 leave-one-out runs on the 'wheel-interaction database'. We also perform the training/testing on the same video: a representative set of video segments is selected from the first 30 min of each video for training; testing is carried out on the remaining of the video from the 30th minute to the end of the same video. System accuracy is computed as a function of the amount of video data (in minute) used for training. ( d ) Average accuracy and standard error across the 13 runs on the 'wheel-interaction database'. Full size image Characterizing the home-cage behaviour of mouse strains To demonstrate the applicability of this vision-based approach to large-scale phenotypic analysis, we characterized the home-cage behaviour of four strains of mice, including the wild-derived strain CAST/EiJ, the BTBR strain, a potential model of autism [4] , as well as two of the most popular inbred mouse strains C57BL/6J and DBA/2J. We video recorded n =7 mice of each strain during one 24-h session, encompassing a complete light–dark cycle. An example of an ethogram containing all the eight behaviours obtained over a 24-h continuous recording period for one of the CAST/-EiJ (wild-derived) strains is shown in Figure 2h . One obvious feature was that the level of activity of the animal decreased significantly during the day (12–24 h) as compared with night time (0–12 h). In examining the hanging and walking behaviours of the four strains, we noted a dramatic increase in activity of CAST/EiJ mice during the dark phase, which show prolonged walking ( Fig. 5a ) and a much higher level of hanging activity ( Fig. 5b ) than any of the other strains tested. Compared with CAST/EiJ mice, the DBA/2J strain showed an equally high level of hanging at the beginning of the dark phase but this activity quickly dampened to that of the other strains, C57BL/6J and BTBR. We also found that the resting behaviour of this CAST/EiJ strain differed significantly from the others: whereas all four strains tended to rest for the same total amount of time (except BTBR, which rested significantly more than C57BL/6J), we found that CAST/EiJ tended to have resting bouts (a continuous duration with one single label) that lasted almost three times longer than those of any other strain ( Fig. 6a,b ). 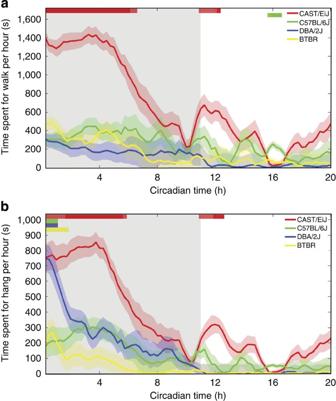Figure 5: Walking and hanging behaviours for the four mouse strains. Average time spent for (a) the 'walking' and (b) 'hanging' behaviours for each of the four strains of mice (n=7 animals for each strain) over a 20-h period. The plots begin at the onset of the dark cycle, which persists for 11 h (indicated by the grey region), followed by 9 h of the light cycle. At every 15 min of the 20-h period, we computed the total time one mouse spent walking or hanging within a 1-h temporal window centred at that current time point. The CAST/EiJ (wild-derived) strain is much more active than the other three strains, as measured by their walking and hanging behaviours. Shaded areas around the curves correspond to 95% confidence intervals and the darker curve corresponds to the mean. The coloured bars indicate the duration when one strain exhibits a statistically significant difference (P<0.01 by analysis of variance with Tukey'spost hoctest) with other strains. Figure 5: Walking and hanging behaviours for the four mouse strains. Average time spent for ( a ) the 'walking' and ( b ) 'hanging' behaviours for each of the four strains of mice ( n =7 animals for each strain) over a 20-h period. The plots begin at the onset of the dark cycle, which persists for 11 h (indicated by the grey region), followed by 9 h of the light cycle. At every 15 min of the 20-h period, we computed the total time one mouse spent walking or hanging within a 1-h temporal window centred at that current time point. The CAST/EiJ (wild-derived) strain is much more active than the other three strains, as measured by their walking and hanging behaviours. Shaded areas around the curves correspond to 95% confidence intervals and the darker curve corresponds to the mean. The coloured bars indicate the duration when one strain exhibits a statistically significant difference ( P <0.01 by analysis of variance with Tukey's post hoc test) with other strains. 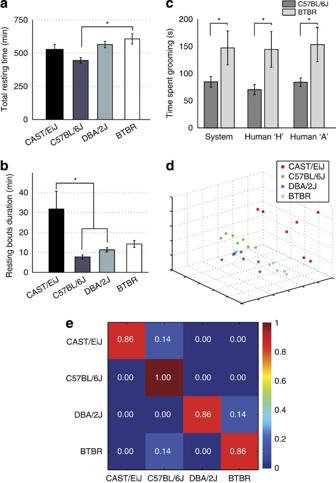Figure 6: Behavioural characterization of four mouse strains. (a) The average total resting time for each of the four strains of mice over 24 h (n=7 animals for each strain). (b) Average duration of resting bouts (defined as a continuous duration with one single behaviour). Values of mean ± s.e.m. are shown, *P<0.01 by analysis of variance with Tukey'spost hoctest. (c) Total time spent grooming exhibited by the BTBR strain as compared with the C57BL/6J strain within 10–20 min after placing the animals in a novel cage. Values of mean±s.e.m. are shown, *P<0.05 by Student'st-test, one-tailed.P=0.04 for system andP=0.0254 for human 'H',P=0.0273 for human 'A'). (d,e) Characterizing the genotype of individual animals on the basis of the patterns of behaviour measured by the computer system. The pattern of behaviours for each animal is a 32-dimensional vector, corresponding to the relative frequency of each of the eight behaviours of interest, as predicted by the system, over a 24-h period. (d) Principal component analysis to visualize the similarities/dissimilarities between patterns of behaviours exhibited by all 28 individual animals (seven mice×four strains). (e) Confusion matrix for a Support Vector Machine (SVM) classifier trained on the patterns of behaviour using a leave-one-animal-out procedure. The SVM classifier is able to predict the genotype of individual animals with an accuracy of 90% (chance level is 25% for this four-class classification problem). The confusion matrix shown here indicates the probability for an input strain (along the rows) to be classified, on the basis of its pattern of behaviour, as each of the four alternative strains (along the columns). The higher probabilities along the diagonal and the lower off-diagonal values indicate successful classification for all categories. For example, the value of 1.0 for the C57BL/6J strain means that all C57BL/6J animals were correctly classified as such. Full size image Figure 6: Behavioural characterization of four mouse strains. ( a ) The average total resting time for each of the four strains of mice over 24 h ( n =7 animals for each strain). ( b ) Average duration of resting bouts (defined as a continuous duration with one single behaviour). Values of mean ± s.e.m. are shown, * P <0.01 by analysis of variance with Tukey's post hoc test. ( c ) Total time spent grooming exhibited by the BTBR strain as compared with the C57BL/6J strain within 10–20 min after placing the animals in a novel cage. Values of mean±s.e.m. are shown, * P <0.05 by Student's t -test, one-tailed. P =0.04 for system and P =0.0254 for human 'H', P =0.0273 for human 'A'). ( d , e ) Characterizing the genotype of individual animals on the basis of the patterns of behaviour measured by the computer system. The pattern of behaviours for each animal is a 32-dimensional vector, corresponding to the relative frequency of each of the eight behaviours of interest, as predicted by the system, over a 24-h period. ( d ) Principal component analysis to visualize the similarities/dissimilarities between patterns of behaviours exhibited by all 28 individual animals (seven mice×four strains). ( e ) Confusion matrix for a Support Vector Machine (SVM) classifier trained on the patterns of behaviour using a leave-one-animal-out procedure. The SVM classifier is able to predict the genotype of individual animals with an accuracy of 90% (chance level is 25% for this four-class classification problem). The confusion matrix shown here indicates the probability for an input strain (along the rows) to be classified, on the basis of its pattern of behaviour, as each of the four alternative strains (along the columns). The higher probabilities along the diagonal and the lower off-diagonal values indicate successful classification for all categories. For example, the value of 1.0 for the C57BL/6J strain means that all C57BL/6J animals were correctly classified as such. Full size image As BTBR mice have been reported to hypergroom [4] , we next examined the grooming behaviour of BTBR mice. In the study by McFarlane et al . [4] , grooming was scored manually during a 10-min session starting immediately after a 10-min habituation period following the placement of the animal in the new environment. Under the same conditions, our system detected that the BTBR strain spent approximately 150 s grooming compared with C57BL/6J mice, which spent a little more than 85 s grooming ( Fig. 6c ). This behavioural difference was reproduced by two more human observers ('H' and 'A') who scored the same videos ( Fig. 6c ). Using annotator 'H' as the ground truth, the frame-based accuracy of the system versus annotator 'A' was 90.0% versus 91.0%. This shows that the system can reliably identify grooming behaviours with nearly the same accuracy as a human annotator. Note that in this study C57BL/6J mice were approximately 90 days old (± 7 days), whereas BTBR mice were approximately 80 days old (± 7 days). In the McFarlane et al . [4] study, younger mice were used (and repeated testing was performed), but our results essentially validate their findings. Prediction of strain type based on behaviour We characterized the behaviour of each mouse with a 32-dimensional vector called the 'pattern of behaviour', corresponding to the relative frequency of each of the eight behaviours of interest, as predicted by the system, over a 24-h period. To visualize the similarities/dissimilarities between patterns of behaviours exhibited by all 28 individual animals (7 mice × 4 strains) used in our behavioural study, we performed a principal component analysis. Figure 6d shows the resulting 28 data points, each corresponding to a different animal, projected onto the first three principal components. Individual animals tend to cluster by strains even in this relatively low-dimensional space, suggesting that different strains exhibit unique patterns of behaviour that are characteristic of their strain types. To quantify this statement, we trained and tested a linear SVM classifier directly on these patterns of behaviour. Figure 6e shows a confusion matrix for the resulting classifier that indicates the probability with which an input strain (along the rows) was classified as each of the four strains (along the columns). The higher probabilities along the diagonal and the lower off-diagonal values indicate successful classification for all strains. Using a leave-one-animal-out procedure, we found that the resulting classifier was able to predict the strain of all animals with an accuracy of 90%. Application of the system to additional mouse behaviours We next asked whether the proposed system could be extended to the recognition of additional behaviours beyond the eight standard behaviours described above. We collected a new set of videos for an entirely new set of behaviours corresponding to animals interacting with 'low profile' running wheels ( Fig. 7a ). The 'wheel-interaction database' contains 13 fully annotated 1-h-long videos taken from six C57BL/6J mice. Here, we consider four actions of interest: 'running on the wheel' (defined by having all four paws on the wheel, with the wheel rotating), 'interacting with the wheel but not running' (any behaviour on the wheel other than running), 'awake but not interacting with the wheel' and 'resting outside the wheel'. Using the same leave-one-video-out procedure and accuracy formulation, as used before for the 'full database', the system achieves 93% accuracy. 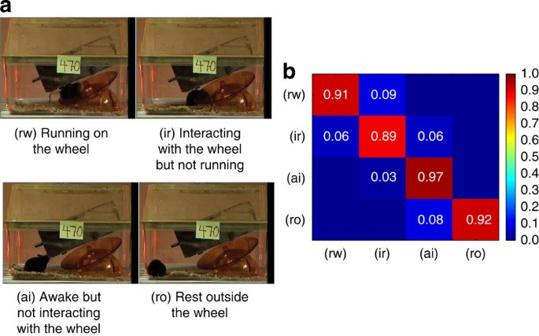Figure 7: Extension of the system to wheel running and investigatory behaviours. (a) Snapshots taken from the 'wheel-interaction database' for the four types of interaction behaviours of interest: resting outside the wheel, awake but not interacting with the wheel, running on the wheel and interacting with (but not running on) the wheel. (b) Confusion matrices for the system (column) versus human scoring (row). The confusion matrix shown in Figure 7b indicates that the system can discriminate between visually similar behaviours, such as 'interacting with the wheel but not running' and 'running on the wheel' (see also Supplementary Movie 3 for a demonstration of the system scoring the wheel-interaction behaviours). To understand how many annotated examples are required to reach this performance, we repeated the same experiment, each time varying the number of training examples available to the system. Data presented in Figure 4c suggest that satisfactory performance can be achieved with only 2 min of annotation for each training video, corresponding to 90% of the performance obtained using 30 min of annotations. Figure 4d shows that training with very short segments collected from a single video seems sufficient for robust performance on the 'wheel-interaction database', but, unlike for the eight standard home-cage behaviours, the system performance increases linearly with the number of training examples. This might be due to the large within-class variation of the action 'awake but not interacting with wheel', which combines all actions that are performed outside the wheel, such as walking, grooming, eating and rearing, within one single category. Figure 7: Extension of the system to wheel running and investigatory behaviours. ( a ) Snapshots taken from the 'wheel-interaction database' for the four types of interaction behaviours of interest: resting outside the wheel, awake but not interacting with the wheel, running on the wheel and interacting with (but not running on) the wheel. ( b ) Confusion matrices for the system (column) versus human scoring (row). Full size image Here we describe a trainable computer vision system capable of capturing the behaviour of a single mouse in the home-cage environment. As opposed to previous proof-of-concept computer vision studies [22] , [23] , our system has been used in a 'real-world' application, characterizing the behaviour of several mouse strains and discovering strain-specific features. Moreover, we demonstrate that this system adapts well to more complex environments and behaviours that involve additional objects placed in the home cage. We provide open-source software and large annotated video databases with the hope that it may further encourage the development and benchmarking of similar vision-based systems. Genetic approaches to understand the neural basis of behaviour require cost effective and high-throughput methodologies to find aberrations in normal behaviours [30] . From the manual scoring of mouse videos (see 'full database' above), we have estimated that it requires approximately 22 person-hours to manually score every frame of a 1-h video with high stringency. Thus, we estimate that the 24-h behavioural analysis conducted above with our system for the 28 animals studied would have required almost 15,000 person-hours of manual scoring. An automated computer vision system permits behavioural analysis that would simply be impossible using manual scoring by a human experimenter. By leveraging recent advances in graphics processing hardware and exploiting the high-end graphical processing units available on modern computers, the current system runs in real time. In principle, our approach should be extendable to other behaviours such as dyskinetic movements in the study of Parkinson's disease models or seizures for the study of epilepsy, as well as social behaviours involving two or more freely behaving animals. In conclusion, our study shows the promise of learning-based and vision-based techniques in complementing existing approaches towards a quantitative phenotyping of complex behaviour. Mouse strains and behavioural experiment All experiments involving mice were approved by the Massachusetts Institute of Technology (MIT) and Caltech committees on animal care. For generating training and testing data, we used a diverse pool of hybrid and inbred mice of varying size, age, gender and coat colour (both black and agouti coat colours). In addition, we varied the lighting angles and used both 'light' and 'dark' recording conditions (with a 30 W bulb dim red lighting to allow our cameras to detect the mice but without substantial circadian entrainment effects.) A JVC digital video camera (GR-D93) with frame rate 30 fps was connected to a PC workstation (Dell) by means of a Hauppauge WinTV video card. Using this setup, we collected more than 24 distinct MPEG-2 video sequences (from one to several hours in length) used for training and testing the system. For processing by the computer vision system, all videos were downsampled to a resolution of 320×240 pixels. The throughput of the system could thus be further increased by video recording four cages at a time using a two-by-two arrangement with a standard 640×480 pixel VGA video resolution. Videos of the mouse strains ( n =28 videos) were collected separately for the validation experiment, using different recording conditions (recorded in a different mouse facility). All mouse strains were purchased from the Jackson Laboratory, including C57BL/6J (stock 000664), DBA/2J (000671), CAST/EiJ (000928) and BTBR T+tf /J (002282). Mice were singly housed for 1–3 days before being video recorded. On the recommendation of Jackson Laboratories, CAST/EiJ mice ( n =7) were segregated from our main mouse colony and housed in a quiet place where they were only disturbed for husbandry 2–3 times per week. This may have influenced our behavioural measurements, as the other three mouse strains were housed in a different room. The mice used for the running wheel study were 3-month-old C57BL/6J males also obtained from Jackson Laboratories. Data annotation Training videos were annotated using a freeware subtitle-editing tool, Subtitle Workshop by UroWorks (available at http://www.urusoft.net/products.php?cat=sw&lang=1 ). A team of eight investigators ('Annotator group 1') were trained to annotate eight typical mouse home-cage behaviours. The four annotators in the 'Annotator group 2' were randomly selected from the 'Annotator group 1' pool. Behaviours of interest included drinking (defined by the mouse's mouth being juxtaposed to the tip of the drinking spout), eating (defined by the mouse reaching and acquiring food from the food bin), grooming (defined by the forelimbs or hindlimbs sweeping across the face or torso, typically as the animal is reared up), hanging (defined by grasping of the wire bars with the forelimbs and/or hindlimbs, with at least two limbs off the ground), rearing (defined by an upright posture and forelimbs off the ground), resting (defined by inactivity or nearly complete stillness), walking (defined by ambulation) and micromovements (defined by small movements of the animal's head or limbs). For the 'full database' to be annotated, every hour of video took about 22 h of labour for a total of 264 h of work. For the 'clipped database', it took approximately 110 h (9 h/h of video) to manually score 9,600 clips of a single behaviour (corresponding to 5.4 h of clips compiled from around 20 h of video). We performed secondary screening to remove ambiguous clips, leaving 4,200 clips for which the human-to-human agreement is very close to 100%. This second screening took around 25 h for the 2.5-h-long 'clipped database'. Supplementary Figures S1a–b and Supplementary Figures S1c–d show the distribution of labels for the 'clipped database' and the 'full database', respectively. Training and testing the system The evaluation on the 'full database' and 'set B' shown in Table 1 was obtained using a leave-one-out cross-validation procedure. This consists of using all but one of the videos to train the system and using the video left out to evaluate the system, repeating this procedure n =12 times for all videos. System predictions for all the frames are then concatenated to compute the overall accuracy as (total number of frames correctly predicted by the system)/(total number of frames) and the human-to-human agreement as (total number of frames correctly labelled by 'Annotator group 2')/(total number of frames). Here, a prediction or label is considered 'correct' if/when it matches the annotations generated by the 'Annotator group 1'. Such a procedure provides the best estimate of the future performance of a classifier and is standard in computer vision. This guarantees that the system is not just recognizing memorized examples but generalizing to previously unseen examples. For the 'clipped database', a leave-one-video-out procedure is used whereby clips from all except one video are used to train the system and testing is performed on clips of the remaining video. This procedure is repeated n =12 times for all videos. A single prediction is obtained for each clip (each clip has a single annotated label) by voting across frames, and predictions for all the clips of all videos are then concatenated to compute the overall accuracy as (number of total clips corrected predicted by the system)/(number of total clips). In addition to measuring the overall performance of the system as above, we also used a confusion matrix to visualize the system's performance on each behavioural category in Figures 3, 6e and 7b . A confusion matrix is a common visualization tool used in multiclass classification problems [23] . Each row of the matrix represents a true class, and each column represents a predicted class. Each entry ( x , y ) in the confusion matrix is the probability that an instance of label x (along the rows) will be classified as instance of label y (along the columns), as computed by (number of instances annotated as type x and classified as type y )/(number of instances annotated as type x ). Here, the frame predictions are obtained by concatenating the predictions for all videos, as described above. The higher probabilities along the diagonal and the lower off-diagonal values indicate successful classification for all behavioural types. For example, in Figure 3a , 94% of the frames annotated as 'rest' are classified correctly by the system, and 5% are misclassified as 'groom'. Comparison with the commercial software To compare the proposed system with available commercial software, the HomeCageScan 2.0 (CleverSys Inc.), we manually matched the 38 output labels from the HomeCageScan to the eight behaviours used in the present work. For instance, actions such as 'slow walking', 'walking left' and 'walking right' were all reassigned to the 'walking' label to match against our annotations. With the exception of very few behaviours (e.g., 'jump', 'turn' and 'unknown behaviour'), we were able to match all HomeCageScan output behaviours to one of our eight behaviours of interest (see Supplementary Table S2 for a listing of the correspondences used between the labels of the HomeCageScan and our system). It is possible that further fine-tuning of HomeCageScan parameters could have improved upon the accuracy of the scoring. Statistical analysis To detect differences among the four strains of mice, analysis of variances were conducted for each type of behaviour independently and Tukey's post hoc test was used to test pairwise significances. All post hoc tests were Bonferroni corrected for multiple comparisons. For the grooming behaviour, a one-tailed Student's t -test was used, as only two groups (C57BL/6J and BTBR) were being compared and we had predicted that BTBR would groom more than C57BL/6J. Mouse strain comparisons Patterns of behaviour were computed from the system output by segmenting the system predictions for a 24-h video into four non-overlapping 6-h-long segments (corresponding to the first and second halves of the day and night periods) and calculating a histogram for the eight types of behaviour for each video segment. The resulting eight-dimensional (one dimension for each of the eight behaviours) vectors were then concatenated to obtain a single 32-dimensional vector (eight dimensions × four segments) for each animal. To visualize the data, we performed a principal component analysis directly on these 32-dimensional vectors. In addition, we conducted a pattern classification analysis on the patterns of behaviour by training and testing an SVM classifier directly on the 32-dimensional vectors. This supervised procedure was conducted using a leave-one-animal-out approach, whereby 27 animals were used to train a classifier to predict the strain of the remaining animal (CAST/EiJ, BTBR, C57BL/6J or DBA/2J). The procedure was repeated 28 times (once for each animal). Accuracy measures for the four strain predictions were then computed as (number of animals correctly classified)/(number of animals). How to cite this article: Jhuang, H. et al . Automated home-cage behavioural phenotyping of mice. Nat. Commun. 1:68 doi: 10.1038/ncomms1064 (2010).